Agronomic conditions and crop evolution in ancient Near East agriculture The appearance of agriculture in the Fertile Crescent propelled the development of Western civilization. Here we investigate the evolution of agronomic conditions in this region by reconstructing cereal kernel weight and using stable carbon and nitrogen isotope signatures of kernels and charcoal from a set of 11 Upper Mesopotamia archaeological sites, with chronologies spanning from the onset of agriculture to the turn of the era. We show that water availability for crops, inferred from carbon isotope discrimination (Δ 13 C), was two- to fourfold higher in the past than at present, with a maximum between 10,000 and 8,000 cal BP. Nitrogen isotope composition ( δ 15 N) decreased over time, which suggests cultivation occurring under gradually less-fertile soil conditions. Domesticated cereals showed a progressive increase in kernel weight over several millennia following domestication. Our results provide a first comprehensive view of agricultural evolution in the Near East inferred directly from archaeobotanical remains. The study of how growing conditions, farming practices and crop domestication evolved from the beginning of agriculture is crucial for revealing the complexity and dynamics of ancient societies and to understand the current Mediterranean landscapes. The initial steps towards plant domestication in the Fertile Crescent can be pushed back to the 12th millennium cal BP, with different cereals being the main staples. Plant domestication in this region was a slow process with crop cultivation appearing at least 1,000 years before the earliest morphological changes supporting domestication (for example, changes in seed shedding, increase in kernel size) [1] . However, the evolution of agricultural systems after domestication, including water availability, soil fertility and potential yields achieved, as well as the pace of ‘post-domestication’ progress in kernel size, remains mostly unknown [2] . The carbon isotope discrimination (Δ 13 C) of charred kernels has been used to reconstruct water conditions [3] , including cereal water inputs of Neolithic [4] , [5] and Bronze Age sites [6] , [7] in the Near East. The comparison of Δ 13 C values from cultivated plant remains (charred seeds) and forest trees (charcoal) has aided the discrimination between climate and anthropogenic effects on crop performance [3] , [8] . Since water availability is the main factor limiting cereal productivity in Mediterranean conditions and, in turn, the Δ 13 C of plant biomass integrates water conditions during growth [9] , information on potential crop productivity can be gained by combining 13 C signatures [10] and kernel weight [11] . Shortages of soil nutrients probably constituted important constraints on growth in prehistoric agriculture [12] . Measures to enhance the availability of nutrients for crops included burning of native vegetation and application of nutrient-enriched sediments, domestic waste, and green and animal manure [13] . However, there is very little direct evidence relating to the history of ancient manuring. Intensive manuring may be taken as an indicator of marked social changes in land use and tenure during the Neolithic [14] . Manuring crops involves a long-term investment in arable land associated with adoption of a sedentary way of life. In general, any agronomic practice aiming to improve soil fertility, such as the use of animal and green manure or fallow, would increase the nitrogen isotope composition ( δ 15 N) of both soil and plants. Different studies suggest that the long-term application of manure to permanently cultivated sites leaves a recognizable N-isotopic imprint on kernels and straw [15] . However, analysis of δ 15 N in kernels as a proxy to infer soil management practices and fertility in ancient agriculture is only a recent development [4] , [11] , [14] , [15] . Kernel weight is a key factor determining nutritional quality in cereals and, as such, has profound economic implications [1] . Archaebotanists interested in the evolution of kernel size at the origin of agriculture usually report on the breadth and thickness of charred kernels [1] . However, kernel dimensions may suffer alterations because of carbonization. Alternatively, the original weight of kernels can be inferred from archaeological (charred) kernel dimensions, after considering the impact of carbonization on three-dimensional deviations [5] , [11] . This allows data of archaeological kernels to be compared with the huge amount of information available on kernel weight for present-day agriculture. Three main objectives were pursued in this study. The first was to characterize the evolution of water availability and nutritional status of cereal crops in the Near East from the beginnings of agriculture to the turn of the era. Second, the increase in kernel weight (ultimately linked to directional selection) was tracked to determine when values comparable to those of present-time cereals were achieved by domesticated barley and naked wheat. Finally, the third objective was to estimate cereal yields in the past as compared with current values for rainfed agriculture in the region. The study shows crop water availability, inferred from Δ 13 C, being two- to fourfold higher in the past than at present, with a maximum between 10,000 and 8,000 cal BP, whereas grain yield values are comparable to those achieved now-a-days in the region. The decrease of δ 15 N over time suggests cultivation occurring under gradually less-fertile soil conditions. A progressive increase in kernel weight over several millennia following domestication is also accounted. Studied kernels Size, δ 15 N and Δ 13 C of charred kernels from five cereal species (including wild and domesticated) ( Supplementary Fig. 1 ), together with charcoal Δ 13 C records of two forest trees ( Quercus sp. and Pistacia sp. ), were studied. These remains belong to a set of 11 Near East archaeological sites (from Upper Mesopotamia or Al-Jazira) spanning 11,000 years from the onset of agriculture in the region (13th millennium cal BP) ( Fig. 1 ). 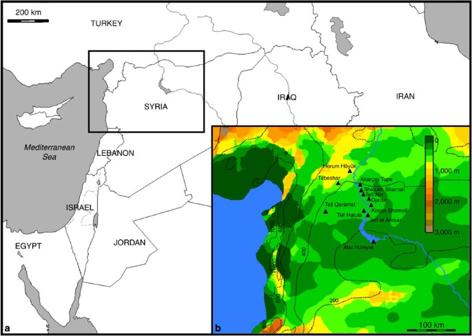Figure 1: Geographical location of the set of 11 Near East archaeological sites where samples were collected. (a) General situation in Upper Mesopotamia. (b) Identification of sites: Abu Hureyra (Epi-Palaeolithic), Akarçay Tepe (middle PPNB/Pre-Halaf), Dja’de (PPNA/Early PPNB), Horum Höyük (Bronze Age), Jerf El Ahmar (PPNA), Kosak Shamali (Chalcolithic), Shioukh Faouqani (ranging from early Bronze to Roman times), Tell Halula (middle PPNB/Halaf), Tell Qaramel (Epi-Palaeolithic), Tilbeshar (Bronze Age), Tell ’Abr 3 (PPNA). Locations include pre-domestication sites dating from the Epi-Palaeolithic (~\n12,700 cal BP) to the Middle PPNB (up to ~\n9,550 cal BP) and fully agricultural sites. Dotted lines indicate precipitation isohyets. Figure 1: Geographical location of the set of 11 Near East archaeological sites where samples were collected. ( a ) General situation in Upper Mesopotamia. ( b ) Identification of sites: Abu Hureyra (Epi-Palaeolithic), Akarçay Tepe (middle PPNB/Pre-Halaf), Dja’de (PPNA/Early PPNB), Horum Höyük (Bronze Age), Jerf El Ahmar (PPNA), Kosak Shamali (Chalcolithic), Shioukh Faouqani (ranging from early Bronze to Roman times), Tell Halula (middle PPNB/Halaf), Tell Qaramel (Epi-Palaeolithic), Tilbeshar (Bronze Age), Tell ’Abr 3 (PPNA). Locations include pre-domestication sites dating from the Epi-Palaeolithic (~\n12,700 cal BP) to the Middle PPNB (up to ~\n9,550 cal BP) and fully agricultural sites. Dotted lines indicate precipitation isohyets. Full size image Crop water status The Δ 13 C of ancient cereals and trees was significantly higher than present-day values achieved under rain-fed conditions in the region ( Fig. 2 ), which points to the prevalence of a plant environment wetter than the present day. At least for early Neolithic agriculture, cultivation in intensive agricultural gardens may have been prevalent in the area. In fact, the most accepted hypothesis among today’s researchers is that early Neolithic agriculture was based on small-scale horticulture on water-retentive alluvial soils [16] such as those found in the middle Euphrates valley, where most of the study sites are located. Previous results on Δ 13 C, together with the evidence of flax cultivation for the PPNB of Tell Halula (one of the sites included in this study), also support planting in wet areas [17] . Nevertheless, reports on a higher Δ 13 C in charcoal recovered in those Neolithic sites compared with present-time wood samples indicate the prevalence of a more humid natural environment than at present [18] . In contrast, by the end of the Early Bronze Age (~\n4,000 BP) irrigation agriculture was widespread in this region [19] . 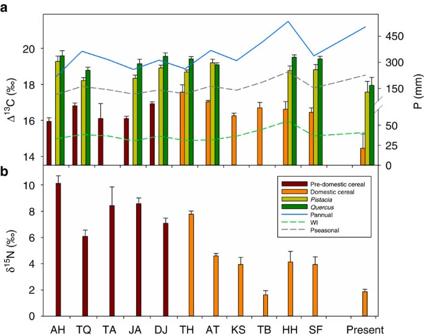Figure 2: Δ13C andδ15N of archaeobotanical samples recovered at each site. (a) Mean values±s.e. of the Δ13C of pre-domestic and domestic cereal kernels andQuercussp. andPistaciasp. charcoal samples recovered at each of the 11 archaeological sites included in this study. Values of present-day samples recovered in the region are included for comparison. (b) Mean values±s.e. ofδ15N of pre-domestic and domestic cereal kernels recovered at each of the 11 archaeological sites included in this study. Values of present-day samples recovered in the region are included for comparison. Abbreviations of the sites and sample sizes (kernels/charcoals) are as follows: Abu Hureyra (AH) (N=9/18), Akarçay Tepe (AT) (N=43/70), Dja’de (DJ) (N=78/27), Horum Höyük (HH) (N=6/43), Jerf El Ahmar (JA) (N=40/43), Kosak Shamali (KS) (N=10/0), Shioukh Faouqani (SF) (N=25/25), Tell Halula (TH) (N=12/88), Tell Qaramel (TQ) (N=17/48), Tilbeshar (TB) (N=11/0), Tell ’Abr 3 (TA) (N=3/0). Present-day kernels correspond to rainfed durum (that is, naked) wheat and barley crops grown in Breda and Boudier (Aleppo, Syria). Present-day values ofQuercusspp. andPistaciaspp. refer to a set of samples collected in the regions of Aleppo and Ar-Raqqah. The lines show the average present-day annual (Pannual), seasonal (Pseasonal) and grain-filling (WI) precipitation at each archaeological site as well as in the sites used to collect present-day kernels and wood samples. Seasonal precipitation was calculated as the precipitation accumulated during the growing period of trees in the region, considered as the interval between March to November. Water input during grain filling of cereals was calculated as the precipitation accumulated during the second half of April plus May. Figure 2: Δ 13 C and δ 15 N of archaeobotanical samples recovered at each site. ( a ) Mean values±s.e. of the Δ 13 C of pre-domestic and domestic cereal kernels and Quercus sp. and Pistacia sp. charcoal samples recovered at each of the 11 archaeological sites included in this study. Values of present-day samples recovered in the region are included for comparison. ( b ) Mean values±s.e. of δ 15 N of pre-domestic and domestic cereal kernels recovered at each of the 11 archaeological sites included in this study. Values of present-day samples recovered in the region are included for comparison. Abbreviations of the sites and sample sizes (kernels/charcoals) are as follows: Abu Hureyra (AH) ( N =9/18), Akarçay Tepe (AT) ( N =43/70), Dja’de (DJ) ( N =78/27), Horum Höyük (HH) ( N =6/43), Jerf El Ahmar (JA) ( N =40/43), Kosak Shamali (KS) ( N =10/0), Shioukh Faouqani (SF) ( N =25/25), Tell Halula (TH) ( N =12/88), Tell Qaramel (TQ) ( N =17/48), Tilbeshar (TB) ( N =11/0), Tell ’Abr 3 (TA) ( N =3/0). Present-day kernels correspond to rainfed durum (that is, naked) wheat and barley crops grown in Breda and Boudier (Aleppo, Syria). Present-day values of Quercus spp. and Pistacia spp. refer to a set of samples collected in the regions of Aleppo and Ar-Raqqah. The lines show the average present-day annual (Pannual), seasonal (Pseasonal) and grain-filling (WI) precipitation at each archaeological site as well as in the sites used to collect present-day kernels and wood samples. Seasonal precipitation was calculated as the precipitation accumulated during the growing period of trees in the region, considered as the interval between March to November. Water input during grain filling of cereals was calculated as the precipitation accumulated during the second half of April plus May. Full size image In the case of barley, the overall agreement between the Δ 13 C of kernels and wood charcoal from the same sites and dating ( Supplementary Fig. 2 ) indicates that water availability through the studied period was mostly determined by the same climatic factors that affected natural vegetation ( Supplementary Note 1 ). In the case of wheat, the Δ 13 C of kernels was not significantly correlated with that of charcoal ( Supplementary Fig. 2 ). Nevertheless, the relationship between the Δ 13 C of wheat and barley became marginally significant ( P =0.08) after samples from one site (Horum Höyük, whose kernels suggest a much better water status for barley) were discarded ( Supplementary Fig. 3 ). Therefore, at least for barley, there is no supporting evidence for an active management strategy aimed at increasing crop water availability (for example, planting in naturally wet areas, water harvesting or even irrigation). The greater water inputs in the past seem to be of climatic origin, a conclusion reinforced by the higher charcoal Δ 13 C of Quercus sp. and Pistacia sp. (species found in open park woodland and woodland steppes, respectively, and not present in riverine forests [20] ) compared with wood samples of these species currently growing in the region ( Fig. 2 ). In fact, barley is now-a-days only cultivated under rain-fed conditions, usually in areas too dry for wheat. Nevertheless, water inputs during grain filling were two- to fourfold higher than today for rain-fed cereals in the region ( Supplementary Fig. 4 ). The wettest period, occurring in the early Holocene between the 11th and 9th millennium cal BP, was immediately preceded by the cool Younger Dryas period (14th–12th millennium cal BP). Water availability at ~\n7th millennium cal BP was lower, thereafter remaining around twice the value of the present time until the turn of the era, but occasionally approaching current values ( Supplementary Fig. 4 ). Crop water inputs matched well with previously reported trends in climate assessed for the region using alternative approaches (see Fig. 3 and references therein). The early Holocene was a period of warming, increases in rainfall and decreases in the amplitude of climatic oscillations. Under these conditions, cultivation probably developed into a sustainable economy. In fact, based on morphometric evidence the earliest domestic cereals identified in this area date to about 10 ka cal BP [21] , [22] . After the climatic optimum of the 11th-10th millennia cal BP, more restrictive water conditions for cultivation, starting at the end of the 9th millennium cal BP, probably coincided with the ‘8.2 ka event’ [23] . Water availability dropped more during the second half of the 5th millennium cal BP, with the lowest estimates coinciding with the ‘4.2 ka event’ [7] . This observation is in line with other studies of Δ 13 C in plant remains reporting increased aridity in the Near East during the Bronze Age [6] , [7] ( Supplementary Note 2 ). Besides this, the existence of local variability in climate effects [24] (for example, upper versus middle Euphrates) ( Supplementary Note 3 ) suggests that aridity was already widespread several centuries before the ‘4.2 ka event’, supporting the drop in Δ 13 C recorded during the mid-Holocene (7–5 ka cal BP). The agreement between kernel Δ 13 C fluctuations and other climate proxies further supports the rainfed nature of cereal cultivation, which was exposed to the vagaries of climate. In addition to climate, low water inputs may also have been related to other factors such as an increasingly greater use of land and cultivation of marginal areas. Expansion into marginal areas has been inferred by archaeologists through observation of changing settlement size [25] . Unlike the Mesopotamian lowlands, which became the focus of irrigation-based riverine civilizations, the settlements of Upper Mesopotamia were primarily based on rainfed agriculture [13] . Even so, our results clearly show that the growing conditions were in general far wetter than for present-time rainfed crops in the region, which supports cultivation during the Neolithic in naturally humid areas and fertile soils [5] . 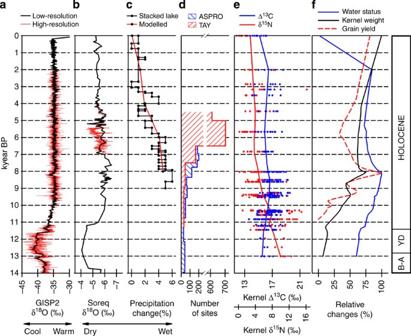Figure 3: Major climatic trends and demographic changes in the region compared with data from the present study. (a) Oxygen isotope composition (δ18O, in ‰) recorded in Greenland ice core GISP2 (refs53,54). More negative values indicate a cooler/drier climate. (b)δ18O in carbonates from Soreq cave in Israel55,56. Lowerδ18O values in cave carbonates are interpreted as being due to higher freshwater inputs and, thus, a wetter climate. (c) Precipitation changes in Eastern Mediterranean (relative to present, in %), according to model simulations57, and stacked and normalized lake isotope record from six lakes in the same region58(d) In blue, the number of sites per period (from ~\n16,000 to 6,500 cal BP), as recorded in the ASPRO Database (http://www.mom.fr/Atlas-des-Sites-du-Proche-Orient.html), including data from sites located in ‘pre-desert’ and ‘steppe’ areas of Syria, Lebanon, Iraq, Turkey, Israel and Palestine. In red, the number of sites per period recorded in the TAY Database (http://www.tayproject.org/enghome.html) for South-Eastern and Eastern Anatolia. Age scale based on average dating of cultural periods in the area (from Pre-Pottery Neolithic to Early Bronze Age, ~\n11,300–4,500 cal. BP). (e) Stable isotope trends in cereal kernels (carbon isotope discrimination, Δ13C, and nitrogen isotope composition,δ15N), including individual data points and locally weighted least-squares regression curves (LOESS) fitted to the data. (f) Summary of modelled trends in the present study: water status, derived from Δ13C in cereal kernels; kernel size, as estimated from kernel dimensions; grain yield, calculated for domestic forms of wheat and barley, from Δ13C and kernel size. Rescaled to relative units, with 0 and 100 standing for the minimum and maximum values of the record, respectively. The bar on the right indicates the major climate periods: B-A, Bølling-Allerød interstadial; YD, Younger Dryas. Radiocarbon calibrated dates obtained from CalPal 2007 (ref.59). Figure 3: Major climatic trends and demographic changes in the region compared with data from the present study. ( a ) Oxygen isotope composition ( δ 18 O, in ‰) recorded in Greenland ice core GISP2 (refs 53 , 54 ). More negative values indicate a cooler/drier climate. ( b ) δ 18 O in carbonates from Soreq cave in Israel [55] , [56] . Lower δ 18 O values in cave carbonates are interpreted as being due to higher freshwater inputs and, thus, a wetter climate. ( c ) Precipitation changes in Eastern Mediterranean (relative to present, in %), according to model simulations [57] , and stacked and normalized lake isotope record from six lakes in the same region [58] ( d ) In blue, the number of sites per period (from ~\n16,000 to 6,500 cal BP), as recorded in the ASPRO Database ( http://www.mom.fr/Atlas-des-Sites-du-Proche-Orient.html ), including data from sites located in ‘pre-desert’ and ‘steppe’ areas of Syria, Lebanon, Iraq, Turkey, Israel and Palestine. In red, the number of sites per period recorded in the TAY Database ( http://www.tayproject.org/enghome.html ) for South-Eastern and Eastern Anatolia. Age scale based on average dating of cultural periods in the area (from Pre-Pottery Neolithic to Early Bronze Age, ~\n11,300–4,500 cal. BP). ( e ) Stable isotope trends in cereal kernels (carbon isotope discrimination, Δ 13 C, and nitrogen isotope composition, δ 15 N), including individual data points and locally weighted least-squares regression curves (LOESS) fitted to the data. ( f ) Summary of modelled trends in the present study: water status, derived from Δ 13 C in cereal kernels; kernel size, as estimated from kernel dimensions; grain yield, calculated for domestic forms of wheat and barley, from Δ 13 C and kernel size. Rescaled to relative units, with 0 and 100 standing for the minimum and maximum values of the record, respectively. The bar on the right indicates the major climate periods: B-A, Bølling-Allerød interstadial; YD, Younger Dryas. Radiocarbon calibrated dates obtained from CalPal 2007 (ref. 59 ). Full size image Soil fertility and manuring Regarding soil fertility, the highest δ 15 N values of archaeological kernels were recorded in the oldest remains, which mostly comprised wild but likely cultivated cereals [26] ( Fig. 2 ). Thereafter, the δ 15 N of both wild and domesticated cereals decreased continuously from the 9th millennium through to the 6th millennium cal BP ( Fig. 4a ). The δ 15 N was in any case much higher than present-time values of wheat and barley for the region, pointing overall to more-fertile conditions in the past. Interestingly, cereals cultivated in the oldest (>10 ka cal BP) versus the most recent (<10 ka cal BP) sites of our study differed in their relationship between Δ 13 C and δ 15 N ( Fig. 4c ). In the oldest sites such an association was lacking, whereas a positive relationship was detected in the more recent sites. This relationship is in line with findings for present-day cereals grown in conditions of limited water availability [11] , [15] , [27] , [28] , indicating that water stress decreases the δ 15 N of plants, and that more-fertile conditions propitiate a better plant water status. A positive relationship was also found between the δ 15 N and N concentration (%) of fossil kernels ( Fig. 4d ). These results support the concept that cultivation under more-fertile conditions (for example, associated with naturally or manure-induced higher δ 15 N) provided an increase in the nutritional qualities (that is, higher protein content) of seeds. Denitrification in wetland or seasonally wet conditions can also lead to high δ 15 N values [29] , [30] . However, this cannot explain the high δ 15 N values at the end of the dry and cold Younger Dryas, and the subsequent decrease during the Early Holocene (see Fig. 3 ). 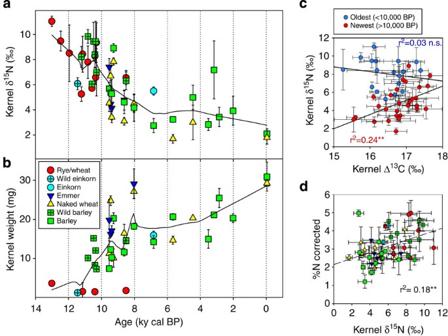Figure 4: Kernel quality and soil fertility. Evolution through time of (a) nitrogen isotope composition (δ15N) and (b) estimated kernel weight of cereal crops. Kernel weight was estimated from the morphometric values of the charred kernels. Trend lines depict locally weighted least-squares regression curves (LOESS) fitted to the data. Each value represents the mean±s.e. of kernels from a specific site and dating. Values for present time kernels as inFig. 2. (c) Relationship betweenδ15N andδ13C of kernels across the oldest (>10 ka cal BP) and the more recent sites. Oldest: Abu Hureyra, Tell Qaramel, Jerf el Ahmar, Tell ’Abr and Dja’de. Newest: other sites. Each point represents the average value for any cereal species, site and dating. (d) Relationship betweenδ15N and the nitrogen concentration in kernels for the set of fossil cereal kernels used in this study. Each point is the mean±s.e. value for a given cereal, dating and site. Figure 4: Kernel quality and soil fertility. Evolution through time of ( a ) nitrogen isotope composition ( δ 15 N) and ( b ) estimated kernel weight of cereal crops. Kernel weight was estimated from the morphometric values of the charred kernels. Trend lines depict locally weighted least-squares regression curves (LOESS) fitted to the data. Each value represents the mean±s.e. of kernels from a specific site and dating. Values for present time kernels as in Fig. 2 . ( c ) Relationship between δ 15 N and δ 13 C of kernels across the oldest (>10 ka cal BP) and the more recent sites. Oldest: Abu Hureyra, Tell Qaramel, Jerf el Ahmar, Tell ’Abr and Dja’de. Newest: other sites. Each point represents the average value for any cereal species, site and dating. ( d ) Relationship between δ 15 N and the nitrogen concentration in kernels for the set of fossil cereal kernels used in this study. Each point is the mean±s.e. value for a given cereal, dating and site. Full size image Alternatively, it has been recently hypothesized that manuring dates back to the initial crystallization of the mixed farming package in western Asia, facilitating the spread of these interdependent practices across diverse climatic zones in Europe [14] . However, in our study the highest δ 15 N was found in pre-domestic cereals, that is, from the oldest sites ( Figs 2 and 4 ), which at first precludes intensive manuring as the cause for such high values. Nevertheless, pre-domestic cultivation does not exclude the possibility of manuring/middening as a management practice ( Supplementary Note 4 ). High δ 15 N in plants may also be a consequence of growing crops in naturally fertile soils, whereas possible environmental factors such as high rainfall and temperature, which could increase δ 15 N, should not be discarded [15] , [28] , at least during the Early Holocene climate optima. The development of early agriculture in soils that were wetter and richer than at present merged with a trend towards cultivation under less favourable conditions with time. A combination of miscellaneous factors of anthropogenic nature (for example, continuous farming, monoculture, diminution of fallow, erosion, cultivation of marginal lands or remoteness from urban centres for efficient manuring), superimposed on a long-term trend of increased aridity, may thus have been involved in the evolution of prehistoric agroecosystems in the Fertile Crescent. The adoption and spread of agriculture set the starting point for significant human-induced impacts on natural ecosystems [31] . Unsustainable practices associated with agricultural overexploitation, such as continuous cultivation (that is, no-fallow farming) together with the use of less fertile soils, were probably present during the Neolithic [5] ( Supplementary Note 5 ). δ 15 N evidence points to decreased soil fertility through to the early Holocene ( Fig. 4 ). However, resource limitation due to land degradation was not likely to occur on a large scale before the Bronze Age [32] . Early Bronze Age (5th and 4th millennium cal BP) urban settlements in Upper Mesopotamia represented a substantial change in scale from Chalcolithic communities (8th and 7th millennium cal BP), with population density, urban places and land-use increasing significantly [13] ( Fig. 3d ). Whether rising population caused land overexploitation, with the consequent degradation of soil fertility, or forced the cultivation of less fertile areas remains a matter for debate. Our results suggest a shift towards more extensive, low-yielding agricultural practices from the Chalcolithic to the Bronze Age, probably balanced with a larger cropping area. Kernel weight Contrasting with the overall trends of environmental degradation, kernel weight increased steadily throughout the Holocene. In addition to the expected changes from pre-domesticated to domesticated cereals ( Fig. 4b ), we found a steep increase until the 10th-8th millennia cal BP, a tendency that continued for several millennia (specially for barley), reaching values similar to present-time rainfed crops in the region ( Fig. 4b ). Our results with domesticated cereals (barley and naked wheat) suggest that kernel weight evolved for a long time after non-shattering ears were present in domesticated wheat and, particularly, barley [1] , [11] . Initial changes in weight may have been favoured by improved environmental conditions for cultivation, that is, phenotypic plasticity [11] . However, this can be discarded as the main driver for the subsequent increase in kernel size, which occurred in parallel with isotopic evidence for impoverished (water and fertility) growing conditions ( Fig. 3f , see also Supplementary Note 6 ). The longer-term trend of change for the first 3,000–4,000 years of agriculture, likely linked to the gradual accumulation of favourable alleles in genes controlling kernel size, points to an evolutionary process affecting domesticated populations [33] . Whereas the kernel weight values used here as the present-time reference for the region are very low (around 30 mg, in accordance with the harsh prevalent rainfed conditions), constitutive values (that is, in the absence of any stress) for both species are around 50 mg or even higher [4] , [28] , [34] . Kernel weight was probably the first trait under artificial selection having a quantitative genetic basis. Because this trait is encoded by multiple genes, its improvement through empirical selection, although feasible, may have been a lengthy process [34] . Nevertheless, historical records show that weights similar to those attained at present were not infrequent [10] , and wheat and barley landraces and old varieties available today exhibit comparable (or even larger) kernel sizes to those of modern cultivars ( Supplementary Note 7 ). Therefore, kernel sizes akin to that of present breeding material were probably achieved a long time ago, but not necessarily during the few millennia after domestication. Following the aforementioned environmental and genetic changes, yield estimates during the Neolithic were in general lower than 0.8 t ha −1 , but showed an increasing trend with time associated with a higher kernel weight up to the 8th millennium cal BP, reaching values of around 1.2 t ha −1 in wheat ( Supplementary Fig. 5 ). Thereafter, yields remained around 0.5 t ha −1 , linked to an increase in aridity until the 6th millennium cal BP. By the 3rd millennium cal BP, yields reached values close to 1 t ha −1 , which are comparable to those currently achieved by rainfed crops in the region [5] , [10] . The estimated yields for ancient cereal agriculture are in line with the historical reports available from the second half of the Holocene and, obviously, do not exclude the occasional occurrence of values several times larger [10] . The minimum cultivated land required per inhabitant in Neolithic sites of the Near East has been estimated to be around 0.25 ha [5] . This value derives from yield estimates of prehistoric agriculture and daily minimum calorie intake [10] and may be extrapolated for later cultural periods in the region (and even considered conservative, considering that productivity probably decreased after the Neolithic) ( Supplementary Fig. 5 ). For a Neolithic settlement like Tell Halula ( Fig. 1 ), with a population fluctuating between ~\n300 and 1,400 inhabitants, the required cultivated land would have ranged between 80 and 700 ha [5] . Although such an estimation of land requirement does not take into account hunting and gathering activities, which may result in lower requirements for land cultivation, small-garden cultivation can be discarded as the only way to grow cereals (the main staples), while suggesting that extensive cultivation was already present during the early stages of agriculture. Moreover, the estimated values are probably in the upper limit range of achievable yields considering breeding advances, water availability and past CO 2 concentrations [35] . Therefore, the above calculation of cultivated land required per inhabitant may be too conservative, which reinforces the conclusion that extensive cultivation was already practised by Neolithic farmers. The existence of much wetter growing conditions in the past compared with present rainfed agriculture agrees with the prevalence of a more humid climate than at present during most of the Holocene in the region ( Fig. 3 ). Moreover, it is believed that the effect of arid periods led to the abandonment of some well-established and large-scale settlements ( Supplementary Note 8 ). Our study shows that the emergence of agriculture in the Fertile Crescent (Upper Mesopotamia) took place under very favourable environmental conditions, provided by wet and fertile soils. However, during the following millennia soil fertility decreased progressively, while water conditions fluctuated in accordance with major climate events and the rainfed nature of cereal crops. Miscellaneous factors such as continuous cultivation, expansion of agricultural practices to less fertile areas or reduced manuring applications may underlie a continuing loss in soil fertility. Despite an overall impoverishment in agronomic conditions, kernel size continued increasing for several millennia after the appearance of domesticated cereal crops as the outcome of a long-term evolutionary process. Archaeobotanical material Agronomic conditions and genetic characteristics of ancient cereal crops, mainly of wheat and barley, were inferred from different traits of charred kernels. A total of 367 cereal kernels and 362 wood remains from 11 sites were analysed. Cereal kernels and wood remains were found in a carbonized state (as charred kernels and charcoal) and were gathered in a disparate manner from domestic fires, cooking ovens and cellar floors. The 729 individual kernels and charcoal fragments were obtained from 245 sediment samples, with a median of five sediment samples per site and dating combination. Soil samples were treated using a standard flotation tank in the field with 0.3 mm (flotation) and 2.5 mm (wet) sieves. Plant remains were then dried slowly before the transport and sorting of seeds. The chronology of archaeobotanical samples was based on stratigraphic dating and radiocarbon ages. All radiocarbon determinations were performed in charcoal samples at Beta Analytic (Miami, Florida, USA). Calibrated ages were determined using the computer program CALIBTH3 (ref. 36 ). The total number and provenance of samples used in this study is summarized in Table 1 . Isotopic data, nitrogen concentration and kernel dimensions (where applicable) of each of the archaeobotanical samples used in this study, as well as the estimated information thus derived (water input, kernel size, grain yield), are also included ( Supplementary Data 1 and 2 ). From the total number of cereal samples, 311 were characterized for stable isotopes and 198 for kernel dimensions. Table 1 Total number of charred kernels and charcoal samples analysed for stable isotopic composition. Full size table Reference material: modern kernels and wood To assess the effect of precipitation on the δ 13 C of modern cereal (durum wheat and barley) and wood material, we selected sampling sites representative of the distribution area of Quercus spp. and Pistacia spp. and of cereal cultivation in the region. Wood cores were obtained for at least five dominant trees per site. For δ 13 C analysis, a fragment of the cores corresponding to the periods 1975–1999 and 1980–2001 was selected for Quercus and Pistacia , respectively. Modern cereal samples came from different experimental trials of the International Center for Agricultural Research in the Dry Areas (ICARDA), as well as from samples collected near the archaeological sites of Tell Halula and Akarçay Tepe. Extended details on the sampling procedure and sample preparation can be found elsewhere [3] , [4] , [8] , [11] , [37] . Stable carbon and nitrogen isotope analyses Carbonate crusts in fossil kernels and charcoal were removed by soaking each kernel and charcoal fragment separately in 6 M HCl for 24 h at room temperature and then rinsing the kernel repeatedly with distilled water [38] . All samples (modern and archaeological) were oven-dried at 60 °C for 24 h before milling to a fine powder for isotope analyses. The stable isotope composition of carbon ( δ 13 C, referred to the VPDB standard) and nitrogen ( δ 15 N, referred to N 2 in air) as well as carbon and nitrogen concentrations (%C, %N) were determined by elemental analysis and isotope ratio mass spectrometry (EA/IRMS) at the Isotope Services of the University of Barcelona (Barcelona, Spain). The overall analytical precision was about 0.1‰ for δ 13 C, 0.2‰ for δ 15 N, 0.6% for %C and 0.1% for %N. Carbon isotope discrimination (Δ 13 C) of archaeobotanical samples was calculated from sample δ 13 C and from the δ 13 C of atmospheric CO 2 , as follows: where δ 13 C air and δ 13 C plant denote air and plant δ 13 C, respectively [39] . The δ 13 C air was inferred by interpolating a range of data from Antarctic ice-core records [40] , [41] , [42] , [43] together with modern data from two Antarctic stations (Halley Bay and Palmer Station) of the CU-INSTAAR/NOAA-CMDL network for atmospheric CO 2 ( ftp://ftp.cmdl.noaa.gov/ccg/co2c13/flask/readme.html ), as described elsewhere [3] , [44] . The whole δ 13 C air data set thus obtained covered the period from 16100 BCE to 2003 CE (data available at http://web.udl.es/usuaris/x3845331/AIRCO2_LOESS.xls ). Charring effects on δ 13 C, δ 15 N and nitrogen concentration Most of the studies available on cereal kernels have reported that δ 13 C [3] , [11] , [44] , [45] and δ 15 N [11] , [46] , [47] are not significantly affected by carbonization within the expected range for carbonization and sample preservation (~\n200–400°C). However, nitrogen concentration in grain is affected by carbonization. Fortunately, the nitrogen concentration of charred kernels can be partly corrected based on the carbon concentration value of the sample [11] . In spite of reports of consistent changes in δ 13 C for ground wood in response to different carbonization treatments [48] , previous results from our team of experimental charring of wood blocks of several species (including the genera Pistacia and Quercus ) have shown negligible shifts in δ 13 C [8] , [45] , [49] . Estimation of kernel weight from charred samples Kernel weight (KW, mg) of wheat and hulled barley can be assessed from the dimensions in mm (length, L; breadth, B; thickness, T) of charred kernels and the level of carbonization [50] , [51] . To get more robust estimates for the different cereal species included, in this study we developed a new model combining data from wheat and barley, according to the following two formulae: Kernel weight was estimated as the mean value of both formulae. The range of grain dimensions and carbonization conditions of this model covered the expected range for the archaeological material. Estimation of water inputs from the Δ 13 C of cereal kernels The Δ 13 C of cereal kernels presents a strong positive relationship with water inputs (precipitation or precipitation plus irrigation) during grain filling across a wide range of Mediterranean conditions [3] , [9] , [45] . We followed the same modelling approach as in earlier studies, but combining data from wheat and barley to obtain a more robust model that could potentially handle other cereal species. Thus, past cereal water inputs (mm) were estimated as follows: As a reference for comparison with present data, total precipitation during grain filling was obtained for the second half of April plus May period [3] , [52] . Estimation of grain yield from Δ 13 C and kernel size Grain yield of cereals was estimated using the model previously developed by our team [10] , [35] . The model takes into account the water status (through the Δ 13 C of kernels), together with changes in Harvest Index (the ratio of kernel weight to total aerial biomass) due to the Green Revolution and the effect of lower-than-present CO 2 (about 270 μl l −1 ) before the Industrial Revolution. Following this [11] , grain yield estimates were further corrected by the smaller kernel size observed in the archaeological kernels when compared with present values (~\n35 mg) in the area [4] , [11] , [50] . Whereas estimated values through this approach probably represent the upper limit range of achievable yields, actual yields were probably lower because of miscellaneous factors such as incidence of weeds, pests and diseases and, in general, poor agronomical conditions. Nevertheless, the advantage of this approach is that it allows estimating yields in a large set of archaeological contexts (wherever seeds are recovered), therefore making it feasible to retrieve information on first agricultural practices, which is obviously not the case for the available written accounts. How to cite this article: Araus, J. L. et al . Agronomic conditions and crop evolution in ancient Near East agriculture. Nat. Commun. 5:3953 doi: 10.1038/ncomms4953 (2014).